Single-molecule fluorescence spectroscopy maps the folding landscape of a large protein Proteins attain their function only after folding into a highly organized three-dimensional structure. Much remains to be learned about the mechanisms of folding of large multidomain proteins, which may populate metastable intermediate states on their energy landscapes. Here we introduce a novel method, based on high-throughput single-molecule fluorescence experiments, which is specifically geared towards tracing the dynamics of folding in the presence of a plethora of intermediates. We employ this method to characterize the folding reaction of a three-domain protein, adenylate kinase. Using thousands of single-molecule trajectories and hidden Markov modelling, we identify six metastable states on adenylate kinase's folding landscape. Remarkably, the connectivity of the intermediates depends on denaturant concentration; at low concentration, multiple intersecting folding pathways co-exist. We anticipate that the methodology introduced here will find broad applicability in the study of folding of large proteins, and will provide a more realistic scenario of their conformational dynamics. Understanding protein folding mechanisms has become a major challenge not only from the viewpoint of basic biological research, but also from that of biomedical studies of diseases caused by misfolding [1] . Analysis of the two-state folding behaviour of small, single-domain proteins [2] , [3] , [4] has led to the suggestion that their folding landscapes (or energy landscapes, that is, the multidimensional surfaces that describe free energy as a function of conformation) were optimized by evolution to be 'smooth', namely to minimize the number of intermediates and/or kinetic traps on the way to the folded state [5] . This might not be the case for larger proteins, especially those built of multiple domains, which constitute more than 70% of the eukaryotic proteome [6] . Past work has already pointed to the possibility that folding of such proteins may involve stable or metastable intermediate states, and classical thermodynamic and kinetic experiments have captured some of this complexity (see, for example, refs 7 , 8 , 9 , 10 , 11 ). Further, spectroscopic methods such as native-state hydrogen exchange have provided detailed structural information on intermediates [12] , [13] . Yet, a particularly daunting task for these experiments has been the characterization of the major kinetic pathways connecting a set of intermediate states. Notably, recent theoretical studies point to the importance of multiple kinetic pathways for folding reactions [14] , even in the case of small proteins [15] . New experimental methods that can readily identify intermediate states and determine their kinetic connectivity are thus much in need. In this work, we demonstrate that single-molecule fluorescence resonance energy transfer spectroscopy (smFRET) [16] , [17] , [18] is well-poised to rise to this challenge. Many smFRET protein folding experiments have been performed on freely diffusing molecules, and have revealed fascinating details on phenomena such as the collapse transition [19] or the nanosecond chain reconfiguration dynamics in the denatured state [20] . However, experiments on freely diffusing molecules are limited to short time scales, of the order of a millisecond, and some form of immobilization is required to study dynamics on longer time scales. Only a handful smFRET folding experiments have been performed on immobilized molecules [21] , [22] , [23] , [24] , [25] . The promise of this type of experiment to identify intermediates in the folding of large proteins and characterize the pathways connecting them [26] has yet to be fulfilled. Here we show how a map of the folding landscape of the three-domain, 214 amino-acid protein adenylate kinase (AK) can be obtained from the analysis of thousands of smFRET trajectories of molecules immobilized within lipid vesicles. AK is a good model protein for such studies. Observation of its structure ( Fig. 1 ) [27] suggests that its three domains interact strongly with each other, and cannot be seen as independent folding units. This picture is reinforced by studies of the intricate functional dynamics of this enzyme, which involve domain closure-type motions [28] , [29] , [30] . Indeed, the complexity of the folding dynamics of AK has been partially unveiled in previous experiments [24] , [31] , [32] , [33] , [34] . Yet, it hasn't been known how many intermediates are involved in AK folding, and what their connectivity is. 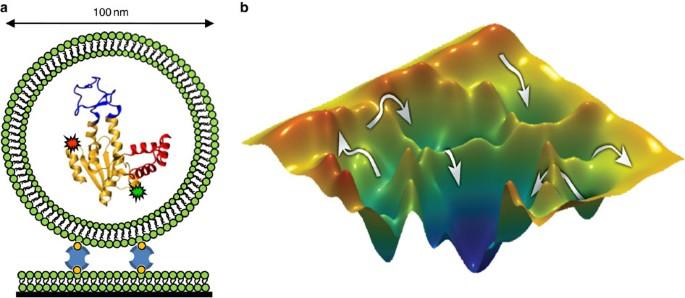Figure 1: Principle of the single-molecule folding experiment. (a) Individual AK molecules, double-labelled for FRET, are encapsulated in vesicles tethered to a glass-supported bilayer using biotin-streptavidin chemistry. The protein molecule is not drawn to scale with the vesicle, which is 100 nm across. (b) In lack of a very long single-molecule temporal trajectory that maps the whole landscape, multiple short trajectories are collected in our experiment. However, the availability of a large number of equilibrium trajectories facilitates reconstruction of the folding landscape using statistical analysis based on HMM. Figure 1: Principle of the single-molecule folding experiment. ( a ) Individual AK molecules, double-labelled for FRET, are encapsulated in vesicles tethered to a glass-supported bilayer using biotin-streptavidin chemistry. The protein molecule is not drawn to scale with the vesicle, which is 100 nm across. ( b ) In lack of a very long single-molecule temporal trajectory that maps the whole landscape, multiple short trajectories are collected in our experiment. However, the availability of a large number of equilibrium trajectories facilitates reconstruction of the folding landscape using statistical analysis based on HMM. Full size image The concept of the experiment reported here is shown in Figure 1 . AK molecules were labelled at positions 73 and 203, which span the CORE domain of the protein [27] . Labelled AK molecules were encapsulated within surface-tethered lipid vesicles ( Fig. 1a ), which provide an excellent means to study single-molecule protein dynamics, as previously shown [24] , [25] , [35] , [36] , [37] , [38] , [39] . Equilibrium experiments were performed in the presence of a series of guanidinium chloride (GdmCl) concentrations, selected so as to lower the folding/unfolding barrier and facilitate molecular dynamics that sample the whole folding landscape of the protein. Thousands of short trajectories were obtained, which, because of the random initial state of each molecule, sampled different regions of the folding landscape of the protein ( Fig. 1b ). Statistical analysis, using hidden Markov modelling (HMM) [40] , then allowed us to effectively 'connect' the trajectories and obtain a single multi-state map of the folding landscape of AK. Single-molecule FRET trajectories of AK An automated single-molecule spectrometer was constructed to facilitate the collection of large sets of single-molecule trajectories, each corresponding to a particular denaturant concentration. Each trajectory, consisting of the photon arrival times of both donor and acceptor fluorophores, was binned in 50 ms time bins, and the FRET efficiency was calculated bin by bin. The availability of a large number of trajectories allowed us to employ rigorous criteria for data validation. These criteria, described in the Supplementary Methods section, enabled a systematic removal of various artefacts in the data set, such as spurious signal levels due to photophysics of one of the dyes. In addition, we explicitly verified that spectral drifts similar to those found by Chung et al . [23] were not observed in our data (see Supplementary Methods for details). After data selection, more than a thousand valid trajectories remained in most data sets ( Fig. 2a ; Supplementary Fig. S5 for sample trajectories, and Supplementary Table S1 for detailed statistics). To validate the quality of these data sets, we calculated the mean FRET efficiency for each and compared these values with the ensemble denaturation curve of AK, measured using FRET as a reporter. Very good agreement was found between FRET efficiency values obtained from the single-molecule data and bulk measurements ( Fig. 2b ). We further compared the probability distributions of FRET efficiency values with FRET efficiency histograms obtained from a free-diffusion single-molecule experiment ( Fig. 2c ), finding excellent agreement in peak positions and widths. 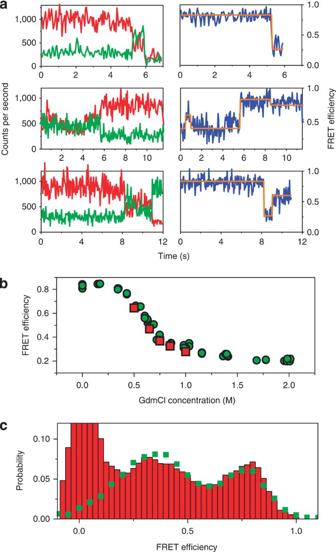Figure 2: Single-molecule FRET trajectories. (a) Three examples of fluorescence trajectories of individual AK molecules, each showing one or more transitions between different FRET efficiency levels. In each example, the left panel shows the experimental traces from the donor and acceptor channels, whereas the right panel shows the FRET efficiency trace, calculated till the photobleaching point. The orange lines in the right panels are state assignments based on the HMM analysis, and obtained with the Viterbi algorithm. The transitions between different FRET states seen in the trajectories are anti-correlated, as were >90% of the transitions seen in our data. See further examples of trajectories inSupplementary Figure S5. (b) Comparison of single-molecule results to the bulk denaturation curve. For the bulk curve, fluorescence spectra of a sample of double-labelled protein molecules were measured at increasing concentrations of GdmCl, and FRET efficiency values were then calculated from them (green points). Single-molecule mean FRET efficiency values (red points) were calculated from the trajectories taken at each GdmCl concentration. These values were obtained by averaging over the initial half a second of each trajectory, so as to avoid the effect of photobleaching. (c) Comparison of the probability distribution of FRET efficiency values obtained from single-molecule trajectories at 0.65 M GdmCl (green squares) to a histogram obtained from a free-diffusion single-molecule experiment performed at the same concentration (red bars). The peak at zero FRET efficiency in the free-diffusion histogram is due to molecules labelled with donor only. Extra FRET efficiency probability distributions appear inFigure 4. Figure 2: Single-molecule FRET trajectories. ( a ) Three examples of fluorescence trajectories of individual AK molecules, each showing one or more transitions between different FRET efficiency levels. In each example, the left panel shows the experimental traces from the donor and acceptor channels, whereas the right panel shows the FRET efficiency trace, calculated till the photobleaching point. The orange lines in the right panels are state assignments based on the HMM analysis, and obtained with the Viterbi algorithm. The transitions between different FRET states seen in the trajectories are anti-correlated, as were >90% of the transitions seen in our data. See further examples of trajectories in Supplementary Figure S5 . ( b ) Comparison of single-molecule results to the bulk denaturation curve. For the bulk curve, fluorescence spectra of a sample of double-labelled protein molecules were measured at increasing concentrations of GdmCl, and FRET efficiency values were then calculated from them (green points). Single-molecule mean FRET efficiency values (red points) were calculated from the trajectories taken at each GdmCl concentration. These values were obtained by averaging over the initial half a second of each trajectory, so as to avoid the effect of photobleaching. ( c ) Comparison of the probability distribution of FRET efficiency values obtained from single-molecule trajectories at 0.65 M GdmCl (green squares) to a histogram obtained from a free-diffusion single-molecule experiment performed at the same concentration (red bars). The peak at zero FRET efficiency in the free-diffusion histogram is due to molecules labelled with donor only. Extra FRET efficiency probability distributions appear in Figure 4 . 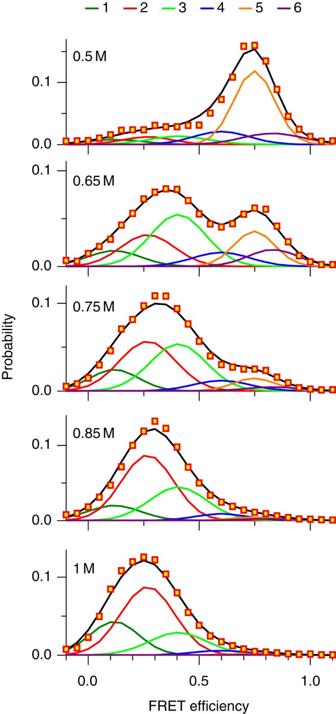Figure 4: State probability distribution histograms, as a function of GdmCl concentration. The probability distributions are based on the parameters extracted from each data set by the HMM analysis. The mean FRET efficiency value of each state was obtained from the analysis of the 0.65 M GdmCl data set, then fixed for analysis of the other data sets. The black lines show the total area-normalized probability distributions, which match very well the distributions calculated directly from the experimental data (yellow symbols). Full size image Change-point analysis of trajectories Using a change-point algorithm, we then analysed each individual trajectory to identify points at which a transition between two FRET efficiency states occurred. The average trajectory length and the average number of transitions per trajectory depended on the GdmCl concentration ( Supplementary Table S1 ), and were 4.3 s and 1.2, respectively, at 0.65 M (close to the denaturation midpoint, Fig. 2b ). The average FRET efficiency change in a transition was 0.18, much smaller than the difference between fully folded and fully unfolded conformations, suggesting that jumps between these conformations are rare. To obtain a global picture of the states visited during folding and unfolding transitions, we used the change-point algorithm to generate a two-dimensional transition map, which plots the transition density as a function of the initial and final FRET efficiency values [24] . Around the denaturation midpoint, a two-state folding reaction should result in a transition map with two peaks symmetrically positioned with respect to the diagonal. The map based on data measured at 0.65 M GdmCl ( Fig. 3a ) deviates significantly from this picture. First, it is not symmetric with respect to the diagonal. This is due to the larger photobleaching rate of the donor probe compared with the acceptor probe, which shortens trajectories that start in more unfolded states (that is, states with lower FRET efficiency). But more importantly, the map shows multiple peaks, each corresponding to a pair of states visited by the molecules as they diffuse on the folding landscape. This is an indication that several intermediate states exist on this landscape. However, the transition map is too dense to resolve and accurately assign all states of the denatured AK, and the situation becomes even more complex at higher concentrations of denaturant, where transitions tend to cluster at lower FRET efficiency values. 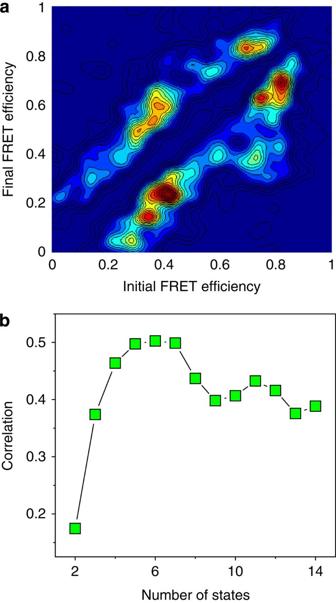Further, a transition map based on change-point analysis does not directly contain information on state-to-state kinetics. Figure 3: Transitions between multiple states in single-molecule trajectories. (a) Transition density map constructed from the 0.65 M GdmCl data set. The map is a two-dimensional density plot of transitions identified by the change-point algorithm, as a function of initial and final FRET efficiencies for each transition. Note the strong deviation of the transition map from that expected for a two-state folder, which should include only two major peaks. (b) Correlation between the transition density map based on change-point analysis and maps based on the HMM analysis with an increasing number of states. The optimal number of states is found to be 5–7. Figure 3: Transitions between multiple states in single-molecule trajectories. ( a ) Transition density map constructed from the 0.65 M GdmCl data set. The map is a two-dimensional density plot of transitions identified by the change-point algorithm, as a function of initial and final FRET efficiencies for each transition. Note the strong deviation of the transition map from that expected for a two-state folder, which should include only two major peaks. ( b ) Correlation between the transition density map based on change-point analysis and maps based on the HMM analysis with an increasing number of states. The optimal number of states is found to be 5–7. Full size image HMM reveals six states To assign the molecular states, as well as the rates of interconversion between them, we employed HMM analysis of the data [40] , [41] . An HMM parses a data set in terms of N discrete states, each presenting a distribution of FRET efficiency values (we take this distribution to be Gaussian). The dynamics of interconversion between these states are assumed to be Markovian. Two important modifications of the standard HMM algorithm were introduced here. First, we required that the dynamics obey detailed balance, so that the flux from any equilibrium state i to any state j equals the inverse flux. Second, we added an extra state, representing the photobleached molecules, and, therefore, connected by a one-way transition to each of the equilibrium states. The introduction of this extra state allowed us to correct for the state-dependent photobleaching rate in a natural way. We used the Baum–Welch algorithm [40] , to obtain a maximum likelihood estimate of the HMM parameters. The analysis was performed on each data set (that is, all trajectories taken at one denaturant concentration) separately. Further details, including error analysis, are given in the Methods section below and in the Supplementary Methods section. As is well known, HMM analysis does not provide an estimate for N . Although various information criteria are sometimes useful for determining N (refs 41 , 42 , 43 ), we devised a different method for this purpose. Focusing on the data set taken at 0.65 M GdmCl (in which the states are expected to be populated most evenly), we repeated the HMM analysis for different values of N , from 2 to 14. We then used the HMM parameters to generate a transition map, and cross-correlated this map with the one obtained from the change-point analysis. The cross-correlation showed that the optimal N is between 5 to 7 ( Fig. 3b ). We therefore used six states for further analysis of all data sets. This method for selecting the number of states was tested against an extensive set of simulations. As a further validation for the number of states, we segmented the trajectories of the 0.65 M GdmCl data set using the Viterbi algorithm, calculated the FRET efficiency value for each segment longer than 1 s, and generated a histogram from all values, shown as Supplementary Figure S6 . Peaks matching the FRET efficiency values of the six states are clearly observed. Since at high GdmCl concentrations states with high FRET efficiencies are rarely visited, we fixed the FRET efficiency value of each state in the analysis, based on the results of the 0.65 M data set, but allowed all other parameters to be optimized by the analysis. State connectivity changes with denaturant concentration Figure 4 shows the FRET efficiency distributions obtained from the HMM analysis. The states are enumerated from 1 to 6 according to their FRET efficiency. At the lowest GdmCl concentration studied, 0.5 M, the distribution is dominated by the population of states with high FRET efficiency. As the GdmCl concentration is increased, states with low FRET efficiency become more and more populated. Observation of transition maps generated from the smFRET trajectories using the HMM parameters ( Fig. 5a–c ) shows that the dynamics of folding and unfolding involve both sequential transitions of the type i → i ±1, and larger, non-sequential transitions of the type i → j , where j > i +1 or j < i −1. Qualitatively, the maps show that with an increasing concentration of GdmCl, the sequential transitions become more dominant. Intriguingly, the most populated state at 0.5 M GdmCl is state 5 rather than state 6. Analysis of the transition maps suggests that state 6 is poorly connected kinetically to state 5, and might be tentatively designated as a misfolded state. Figure 4: State probability distribution histograms, as a function of GdmCl concentration. The probability distributions are based on the parameters extracted from each data set by the HMM analysis. The mean FRET efficiency value of each state was obtained from the analysis of the 0.65 M GdmCl data set, then fixed for analysis of the other data sets. The black lines show the total area-normalized probability distributions, which match very well the distributions calculated directly from the experimental data (yellow symbols). 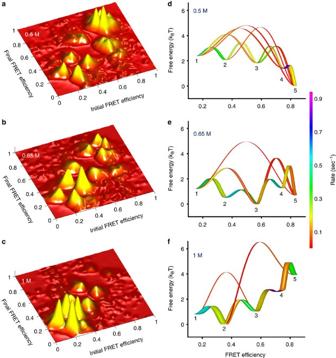Figure 5: The folding landscape of AK. (a–c) Transition maps at three indicated GdmCl concentrations, constructed from the experimental data using HMM analysis results. As the concentration of denaturant increases, more transitions tend to occur between states of lower FRET efficiency. In addition, the fraction of sequential transitions of the typei→i±1increases significantly. (d–f) One-dimensional projections of the folding landscape of AK at the three indicated GdmCl concentrations. State 6, which is poorly connected to state 5, is not shown. The relative free energy of each state was extracted from the probability distributions ofFigure 4. The heights of the free energy barriers between pairs of states were calculated from the HMM transition probability matrices (the value of the pre-exponential factor in the Arrhenius equation was set to 1). Line widths depict the relative productive flux flowing between each pair of states, whereas the colours depict the rate of each transition, according to the scale shown on the right. Only transitions that carry at least 10% of the flux from state 5 to state 1 (or vice versa) are shown. Full size image Figure 5: The folding landscape of AK. ( a – c ) Transition maps at three indicated GdmCl concentrations, constructed from the experimental data using HMM analysis results. As the concentration of denaturant increases, more transitions tend to occur between states of lower FRET efficiency. In addition, the fraction of sequential transitions of the type i→i±1 increases significantly. ( d – f ) One-dimensional projections of the folding landscape of AK at the three indicated GdmCl concentrations. State 6, which is poorly connected to state 5, is not shown. The relative free energy of each state was extracted from the probability distributions of Figure 4 . The heights of the free energy barriers between pairs of states were calculated from the HMM transition probability matrices (the value of the pre-exponential factor in the Arrhenius equation was set to 1). Line widths depict the relative productive flux flowing between each pair of states, whereas the colours depict the rate of each transition, according to the scale shown on the right. Only transitions that carry at least 10% of the flux from state 5 to state 1 (or vice versa) are shown. Full size image 1D projections of the folding landscape of AK at three GdmCl concentrations, based on the HMM parameters, are shown in Figure 5d–f . The relative free energies of states 1–5 are plotted. In addition, the figures also present the heights of the free energy barriers for transitions between pairs of states. For clarity, we show only transitions that carry more than 10% of the unfolding (or folding) flux. These were calculated using either the transition-path theory of Noé et al . [44] or a stochastic simulation, with similar results ( Supplementary Table S2 ). The widths of the lines in Figure 5d–f depict the relative productive flux flowing between each pair of states, and their colours represent the transition rates. At 0.5 M GdmCl, many transitions, both of the sequential and of the non-sequential type, have low enough free energy barriers to participate significantly in unfolding pathways. The unfolding flux thus goes through many parallel pathways. However, when the denaturant concentration is increased to 1 M, most non-sequential transitions have high free energy barriers, and therefore do not contribute significantly to the productive flux. Indeed, ∼ 50% of the unfolding flux is now carried through the fully sequential pathway 5→4→3→2→1 ( Supplementary Table S2 ). Nevertheless, even under these conditions a considerable fraction of the trajectories include larger jumps. The results presented here show that single-molecule FRET spectroscopy can provide a comprehensive description of the folding landscape of a large, multidomain protein like AK in terms of the metastable states involved and the rates of transitions between them. The picture arising is dramatically different and more complex than the usual two-state folding behaviour seen in small proteins, where a single transition state dominates the reaction. Indeed, it is found that the dynamics involve a large set of possible pathways on the landscape. An important feature of the folding landscape of AK is the increasingly more sequential nature of the dynamics with increased denaturant concentration, with a larger and larger share of the flux going through the fully sequential pathway. What is the structural nature of the intermediates identified in our experiment? At this point of time, we refrain from attempting an answer to this question, as only projections of these structures on a single distance were measured in the current work. It is possible that part of the complexity in AK folding can be attributed to proline cis-trans isomerization [45] . Our results are consistent with the work of Haas and co-workers, who demonstrated the complex nature of AK folding in a series of kinetic FRET experiments [33] , [34] , [46] . In particular, these authors found that the distance 73–203 contracts in 2 ms and then presents with a broad distribution that slowly narrows down to that of the native state [46] . This broad distribution may hide the intermediate states seen in our experiment. More generally, the current work is consistent with the foldon picture [13] , [47] , and provides the experimental means to characterize foldon dynamics. However, the dynamics observed here are considerably richer than the simple sequential dynamics suggested by Englander and co-workers [12] , and may vary significantly with experimental conditions. In the future, it will be interesting to combine the results from our smFRET experiment with those obtained from a method like native-state hydrogen exchange, which affords detailed structural information on foldons more readily, but might be lacking in its ability to trace their connectivity and dynamics. Our analysis and results are also likely to offer an important link to simulations that describe protein folding in terms of Markov models [15] , [44] . Indeed, in future work, we plan to combine computer simulations and measurements of further intramolecular distances to obtain more information on the structure of the intermediate states of AK. Protein expression and labelling The expression vector containing the Escherichia coli AK gene was a generous gift from Professor Elisha Haas (Bar-Ilan University). Standard site-directed mutagenesis methods were used to substitute alanines at positions 73 and 203 of the protein with cysteines. The large variation in labelling rate between the two sites [33] facilitated site-specific labelling with Alexa 488 maleimide (Invitrogen) at position 73 and ATTO 590 maleimide (ATTO–TEC) at position 203. More details can be found in the Supplementary Methods section. Sample preparation for single-molecule studies Vesicles made of egg phosphatidylcholine and a fraction of 1:500 of biotynilated phosphoethanolamine (both from Avanti Lipids) were prepared by extrusion [34] in a buffer containing the appropriate concentrations of labelled proteins and chemical denaturant. The glass surfaces of the sample cell were initially coated with a supported bilayer, which contained the same fraction of biotynilated lipids as above. Strepatividin was added, followed by protein-loaded vesicles. Single-molecule setup and data acquisition The sample cell was mounted on top of a capacitance-feedback piezo stage and excited by the focused 488 nm beam of an argon ion laser. The arrival times of fluorescent photons were registered by two single-photon avalanche photo-diodes. Data acquisition was fully automated using dedicated software. A 5 μm×5 μm region of the sample was scanned, and the position of vesicles loaded with molecules was identified with subpixel resolution. The piezo stage was positioned on each of these in turn, to obtain a fluorescence time trace (trajectory). After acquiring trajectories of all molecules in a field, the piezo stage was moved to a new region, and the acquisition cycle was repeated. The laser power was set to 1,000 nW during the scan and 250 nW during time-trace acquisition. An auto-focus device ensured that the laser beam was focused on the surface of the sample throughout data collection. Further details on the experimental setup can be found in the Supplementary Methods section. Data analysis As folding/unfolding transitions in AK are slow (of the order of 1 s), we first binned fluorescence trajectories (accumulated as photon arrival times on the two detectors) in 50 ms time bins. We used a series of computational filters to ensure that only trajectories generated by individual molecules were included in the analysis, and to prevent the occurrence of various artefacts (see Supplementary Methods ). Trajectories that passed the filtration stage were corrected for background and leakage of photons from donor to acceptor channel, which amounted to ∼ 7%. FRET efficiency was calculated for each bin using The factor γ corrects for different quantum efficiencies of the donor and acceptor, as well as different detection efficiencies in the two detection channels. We evaluated γ directly from single-molecule trajectories and found it to be ∼ 1 for our setup. To identify transitions between FRET efficiency levels in a model-independent manner, single-molecule trajectories were subjected to a change-point analysis (see the Supplementary Methods section). Bootstrapped trajectories were used to estimate the statistical significance of identified transitions. More than 90% of the identified transitions involved anti-correlated changes in donor and acceptor channels. The FRET efficiency values of the data segments before and after each transition served as coordinates for a point on a two-dimensional map. Each such point was then dressed with a 2D normalized Gaussian function, which facilitated the construction of transition density maps. HMM analysis of the data assumed a model of Markovian dynamics involving N discrete states, the FRET efficiency of each being normally distributed. For this analysis, we modified a freely-distributed MATLAB toolkit ( http://www.cs.ubc.ca/~murphyk/Software/HMM/hmm.html ). A 'photobleached' state was added to the N states of the basic model, to account for the irreversible signal loss at the end of each trajectory. In practice, this was done by appending a short termination sequence to each trajectory, with an artificially large FRET value. This value made the transition into the termination state effectively irreversible. Multiple random initial conditions were used to start the iterative HMM analysis, to ensure convergence to the global minimum. The Baum–Welch algorithm was used to re-estimate the parameters at the end of each iteration [40] . Detailed balance was enforced on the re-estimated parameters in each iteration based on the condition π i a ij = π j a ji , where a ij is the transition probability from state i to state j per time bin, and π i is the equilibrium probability of state i . In particular, the transition probabilities estimated by the Baum–Welch algorithm were then corrected according to for i ≠ j , and Obviously, only parameters related to the original N states were corrected in this manner. We verified that the enforcement of detailed balance in this fashion did not significantly modify the convergence pattern of the algorithm. In fact, we found that the resulting estimators outperformed the original, non-constrained Baum–Welch estimators when used to analyse simulated data obeying detailed balance. A sample transition probability matrix obtained from the HMM analysis of the 0.65 M GdmCl data set is shown in Supplementary Table S3 . Transition density maps were constructed based on the experimental data and the optimal HMM parameters. In brief, the likelihood of each possible segmentation of each trajectory was computed, and the total likelihood for transition between pairs of FRET efficiency values was calculated by summation over all trajectories. Each such likelihood value was then dressed with a 2D normalized Gaussian function, as in the construction of change-point maps. How to cite this article: Pirchi, M. et al . Single-molecule fluorescence spectroscopy maps the folding landscape of a large protein. Nat. Commun. 2:493 doi: 10.1038/ncomms1504 (2011).